Plasmon-mediated magneto-optical transparency Magnetic field control of light is among the most intriguing methods for modulation of light intensity and polarization on sub-nanosecond timescales. The implementation in nanostructured hybrid materials provides a remarkable increase of magneto-optical effects. However, so far only the enhancement of already known effects has been demonstrated in such materials. Here we postulate a novel magneto-optical phenomenon that originates solely from suitably designed nanostructured metal-dielectric material, the so-called magneto-plasmonic crystal. In this material, an incident light excites coupled plasmonic oscillations and a waveguide mode. An in-plane magnetic field allows excitation of an orthogonally polarized waveguide mode that modifies optical spectrum of the magneto-plasmonic crystal and increases its transparency. The experimentally achieved light intensity modulation reaches 24%. As the effect can potentially exceed 100%, it may have great importance for applied nanophotonics. Further, the effect allows manipulating and exciting waveguide modes by a magnetic field and light of proper polarization. The magneto-optical activity of a magnetized medium is mainly described by its gyration g in the non-diagonal terms of the permittivity tensor [1] . Effects that are quadratic in magnetization M are also determined by the magnetization-induced changes of the diagonal elements of the permittivity tensor (Methods). For materials of cubic symmetry, g is proportional to M . In bulk, these terms lift the degeneracy of electromagnetic modes with respect to light polarization, inducing a splitting between orthogonally circularly or linearly polarized modes. This splitting gives rise to the Faraday or Voigt magneto-optical effects [1] . In a spatially confined medium, the electromagnetic mode structure is more complex. Further, an external magnetic field can modify frequencies and distributions of the modes giving rise to a multifaceted phenomenology [2] , [3] , [4] , [5] . An additional degree of freedom opens up in metal-dielectric nanocomposites [6] , [7] as well as periodic magnetic structures with the period close to the wavelength of a mode [8] , [9] , [10] , [11] , [12] , [13] , [14] , [15] . Periodic structures with metallic and dielectric constituents—plasmonic crystals—can support surface plasmon polaritons along with waveguide modes [16] . Magneto-induced changes of sample transmittance and reflectance due to cyclotron resonance were predicted for plasmonic crystals containing perforated non-magnetic materials with a Drude ac conductivity tensor [17] , [18] . However, this effect requires rather large external magnetic fields exceeding 1 Tesla. Much smaller values of a control magnetic field are feasible if the plasmonic crystal includes magnetic materials, which is referred to as magneto-plasmonic crystal (MPC). Such an MPC provides outstanding magneto-optical properties as evidenced by significant enhancements of the Faraday and transverse Kerr effects [19] , [20] , [21] , [22] , [23] , [24] , [25] , [26] , [27] , [28] , [29] , [30] . The mostly pronounced enhancement of the magneto-optical effects was found for MPCs containing a perforated noble metal stacked on a magnetic dielectric film [27] , [28] , [29] , [30] . Because of their constituents, such MPCs have a large specific Faraday rotation due to the magnetic dielectric and small optical losses due to the nanostructured noble metal. Physical origin of such an enhancement is related to the excitation of the surface plasmon polaritons and waveguide modes of the MPC, which, on the one hand, leads to resonances in the transmittance and reflectance spectra that are sensitive to the magnetic field and, on the other hand, increases the effective length of light interaction with the magnetized medium. Here we demonstrate that apart from enhancing established magneto-optical effects, MPCs can also be used to generate novel phenomena. In particular, we report about a new magneto-photonic effect in the longitudinal magnetization configuration by which the MPC transparency is resonantly increased by about 24%. The effect may be increased even further by using materials with better magneto-optical quality, making it attractive for applications in modern telecommunication devices. Eigenmodes of the MPC We consider an MPC consisting of three layers. From bottom to top the layer sequence is ( Fig. 1a ): a non-magnetic dielectric substrate, followed by a magnetic dielectric layer, and a thin gold film stacked on top. The latter is periodically perforated by parallel slits with period d . The lower refractive index of the substrate relative to one of the magnetic layer ensures the existence of guided optical modes in the magnetic layer. 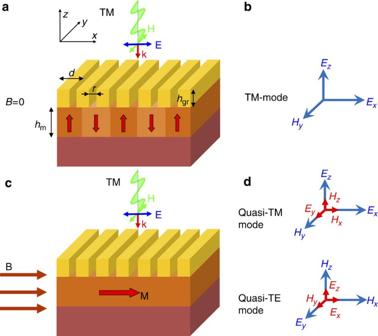Figure 1:Electromagnetic modes of theMPC. (a,c) Schematics of MPCs in (a) demagnetized (multidomain) and (c) longitudinally magnetized conditions. The MPC consists of a gold grating of heighthgrstacked on a smooth ferromagnetic dielectric of thicknesshmgrown on a non-magnetic substrate. The gold grating has perioddand slit widthr. (b,d) Optical modes that can be excited by incident TM-polarized light (Efield is perpendicular to the gold slits) for the (b) demagnetized and (d) longitudinally magnetized structure. The long blue arrows represent the principal field components associated with TM and TE modes in the non-magnetic case, whereas the short red arrows indicate the components induced by the longitudinal magnetization. Figure 1: Electromagnetic modes of the MPC. ( a , c ) Schematics of MPCs in ( a ) demagnetized (multidomain) and ( c ) longitudinally magnetized conditions. The MPC consists of a gold grating of height h gr stacked on a smooth ferromagnetic dielectric of thickness h m grown on a non-magnetic substrate. The gold grating has period d and slit width r . ( b , d ) Optical modes that can be excited by incident TM-polarized light ( E field is perpendicular to the gold slits) for the ( b ) demagnetized and ( d ) longitudinally magnetized structure. The long blue arrows represent the principal field components associated with TM and TE modes in the non-magnetic case, whereas the short red arrows indicate the components induced by the longitudinal magnetization. Full size image In absence of an external magnetic field, the magnetic layer is demagnetized ( Fig. 1a ). Then the eigenmodes hosted by the MPC are surface plasmons as well as waveguided transverse magnetic (TM) or transverse electric (TE) waves. The TM and TE modes are mostly localized in the magnetic layer. Nevertheless, they are (especially the TM mode) sensitive to the permittivity of the adjacent metal and therefore also have plasmonic character. The TM and TE modes have three non-zero field components ( Fig. 1b ) and , respectively. The periodic perforation of the gold layer leads to Bloch wave character of these modes and to their leakage into the surrounding air so that the modes have a significant role for the optical far-field response of the structure. Indeed, these modes cause resonances with non-symmetric Fano-shape in the transmittance T and reflectance R spectra [31] . The TM and TE modes can be excited by the incident light with momentum component if momentum conservation is fulfilled: , where , κ is the mode wavenumber and m is an integer. In addition, the incident light wave must have the proper polarization so that it has at least one component along the electromagnetic field of the mode. For example, a TE mode can be excited only if the incident wave has a E y field component, which is satisfied for TE-polarized illumination ( E field is along the slits). An external DC magnetic field B , applied along the x -axis, magnetizes the magnetic layer of the MPC longitudinally ( Fig. 1c ) so that non-diagonal terms of the tensor appear: ɛ yz =− ɛ zy = ig . Their presence transforms the modes into ‘quasi-TM’ and ‘quasi-TE’ modes ( Fig. 1d ). Besides the TM components, the quasi-TM mode also contains TE components: . Vice versa, the quasi-TE mode acquires TM components: . Because all six field components are non-zero for both modes, those modes can be excited by the incident light of any polarization. For normal incidence of the TM-polarized ( E is perpendicular to the slits) light experimentally studied here, the excited waveguide modes have the E x and H y components of even parity in x , as inherent in the incident radiation. These modes are quasi-TM and quasi-TE ones with the following form of Bloch–Fourier series expansion: where U TM/TE are Fourier amplitudes of Bloch envelopes for principal components of the quasi-TM/quasi-TE modes, F(κ, z) and G(κ, z) are defined by the parameters of the magnetic layer waveguide (Methods). According to equation 1, the admixed components of the modes are proportional to g and, consequently, to the magnetization. The appearance of the admixed field components can also be understood in terms of the TM–TE mode conversion taking place in the longitudinally magnetized waveguide due to the circular birefringence [3] . However, this reasoning becomes cumbersome for the case of a standing wave. Moreover, for symmetry reasons, no transformation of light polarization occurs in the far field for normal incidence. Longitudinal magneto-photonic intensity effect The mode wavenumber of the quasi-ТM and quasi-TE modes in the longitudinally magnetized structure changes according to (Methods): For typical values of g , the shift of Fano resonances induced by these changes is relatively small and therefore would result only in small modifications of the transmittance/reflectance spectra. A considerably larger effect is expected to come from the magnetization-induced changes of the field distributions of the modes. The key point in that respect is that because of the appearance of the TM components in the quasi-TE mode, this mode can be excited by light of TM polarization. The excited quasi-TE mode takes a fraction of the incident optical energy, changing the overall absorbed energy by Δ A . Equation 1 implies that the quasi-TE mode amplitude is proportional to the gyration g . Consequently, Δ A g 2 , and because of energy conservation, the changes in transmittance Δ T and reflectance Δ R are also quadratic in g . For zeroth order of diffraction, the considered magneto-optical intensity effect can be described by the relative difference between the transmittance coefficients T M and T 0 of the magnetized and the demagnetized structure: observed at the TE-mode eigenfrequencies. Because the longitudinal magnetization of the MPC also modifies the field of the TM modes by inducing TE components, one should expect intensity variation at the TM-mode resonances as well. A similarly defined intensity-related effect, but of different origin, was studied in conventional magneto-optics of smooth ferromagnets, and was called orientational effect [32] , [33] . However, for illumination polarized along the magnetization, the orientational effect vanishes [33] . Therefore, the effect considered here has to be regarded as novel, with the most prominent feature being that the effect is exclusively caused by the excitation of eigenmodes of the nanostructured medium so that it may be termed ‘longitudinal magneto-photonic intensity effect’ (LMPIE). Experimental demonstration To provide a proof-of-principle demonstration of the effect, we fabricated several MPCs, and the highest value of the LMPIE is found for the sample based on a 1,270-nm thick magnetic film of composition Bi 2.97 Er 0.03 Fe 4 Al 0.5 Ga 0.5 O 12 , possessing a large real part of gyration g =0.015 and a low absorption coefficient α =400 cm −1 (ref. 34 ) at 840 nm. The other prominent feature of this sample is that it was designed such that the dispersion curves of the principal TM and TE modes corresponding to m =2 intersect at the Г point ( κ =0) of the Brillouin zone. As a consequence, both modes can be excited by normally incident light of the same frequency. The MPC has a gold grating with period d =661 nm, height h gr =67 nm and slit width r =145 nm. The LMPIE was observed in transmission (Methods). Intensities of the zeroth-diffraction-order-transmitted light for demagnetized and longitudinally magnetized MPCs were compared to determine the parameter δ that characterizes the LMPIE. First, we checked that no intensity modulation occurs for the bare magnetic film ( Fig. 2a , green curve). Thereafter, we measured the LMPIE for the MPC illuminated with normally incident TM-polarized light and found that the longitudinally applied magnetic field resonantly increases MPC transparency by 24% at λ =840 nm ( Fig. 2a ). There are also resonances at about 825 and 801 nm, though their values are several times smaller. Numerical modelling results (blue curve in Fig. 2a ) agree closely with the experimental data (Methods). 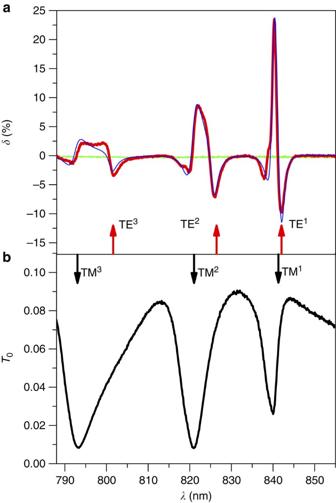Figure 2: Experimentally measured magneto-photonic effect for modulating the intensity of the transmitted light. (a) Spectrum of the LMPIE when a magnetic fieldB=320 mT reaching almost the saturation value is applied. Blue curve shows calculatedδ. There is no LMPIE for the bare magnetic film (green curve). (b) Spectrum of the optical transmittance for the demagnetized structure. Black and red arrows indicate calculated spectral positions of the quasi-TM and quasi-TE resonances, respectively. The modes are denoted by the number of theirHyorEyfield maxima along thezaxis. The light is TM-polarized and hits the sample under normal incidence. All measurements were performed at room temperature. The MPC sample parameters are:d=661 nm,hgr=67 nm,r=145 nm andhm=1,270 nm (seeFig. 1a). Figure 2: Experimentally measured magneto-photonic effect for modulating the intensity of the transmitted light. ( a ) Spectrum of the LMPIE when a magnetic field B =320 mT reaching almost the saturation value is applied. Blue curve shows calculated δ . There is no LMPIE for the bare magnetic film (green curve). ( b ) Spectrum of the optical transmittance for the demagnetized structure. Black and red arrows indicate calculated spectral positions of the quasi-TM and quasi-TE resonances, respectively. The modes are denoted by the number of their H y or E y field maxima along the z axis. The light is TM-polarized and hits the sample under normal incidence. All measurements were performed at room temperature. The MPC sample parameters are: d= 661 nm, h gr =67 nm, r= 145 nm and h m =1,270 nm (see Fig. 1a ). Full size image Properties of the LMPIE The transmittance spectrum demonstrates three Fano resonances clearly related to excitation of TM modes whose spectral positions (shown by the black arrows in Fig. 2b ) were calculated by the scattering-matrix method (see Methods). The calculated spectral positions of the quasi-TE modes indicated by the red arrows in Fig. 2a , on the other hand, confirm that excitation of these modes is responsible for the LMPIE peaks. A longitudinal magnetic field causes almost no shift of the Fano resonances but modifies their shapes substantially. That is why the LMPIE spectral lines have rather complex multiple peak character. An important feature of the designed MPC is that the TE-mode resonance is tuned away from the transmittance minimum, allowing one to simultaneously have high transmittance (see for example, the negative peak of δ =−10.3% at λ =842 nm in Fig. 2a ). The LMPIE shows maximum values of about 24% at λ =840 nm where both quasi-TE and quasi-TM mode resonances are excited. Simultaneous excitation of the two orthogonal modes allows more efficient trapping of the TM-polarized illumination and its conversion into the quasi-TE mode due to the applied magnetic field. This is also supported by the spatial distribution of the E field of the optical wave inside the magnetized MPC, calculated at the two quasi-TE-mode resonances (at 840 and 801 nm) ( Fig. 3a ). Coloured contour plot depicts E y , which is one of the principal field components of the quasi-TE mode. Squares of the quasi-TE-mode amplitude differ by a factor of 14, and the larger the amplitude of the TE-mode, the larger the effect in the far field, that is, the LMPIE. In the case of a demagnetized MPC, the quasi-TE mode vanishes demonstrating the near-field aspect of the LMPIE, that is, switching on and off of the quasi-TE mode by the external magnetic field ( Fig. 3b ). 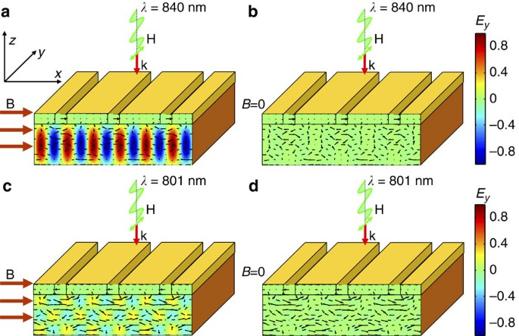Figure 3: Magneto-photonic effect in the optical near field. Calculated spatial distributions of the optical electric field componentEy(shown by the coloured contour plots). The component of the electric field lying in the plane perpendicular to the slitsE||(E||=Exex+Ezez, whereexandezare unit vectors along thexandzaxis, respectively) is shown by arrows. Four cases are presented: (a) longitudinally magnetized MPC at the almost degenerate TM- and TE-mode resonance (atλ=840 nm), (b) demagnetized MPC atλ=840 nm, (c) longitudinally magnetized MPC at the solitary TE resonance (atλ=801 nm) and (d) demagnetized MPC atλ=801 nm. The light hits the sample under normal incidence and is TM-polarized. Parameters of the MPC correspond to the experimentally studied structure. Full magnetization saturation in the external magnetic field is assumed.EyandE||are shown at times when their respective values are maximum. Figure 3: Magneto-photonic effect in the optical near field. Calculated spatial distributions of the optical electric field component E y (shown by the coloured contour plots). The component of the electric field lying in the plane perpendicular to the slits E || ( E || = E x e x + E z e z , where e x and e z are unit vectors along the x and z axis, respectively) is shown by arrows. Four cases are presented: ( a ) longitudinally magnetized MPC at the almost degenerate TM- and TE-mode resonance (at λ =840 nm), ( b ) demagnetized MPC at λ =840 nm, ( c ) longitudinally magnetized MPC at the solitary TE resonance (at λ =801 nm) and ( d ) demagnetized MPC at λ =801 nm. The light hits the sample under normal incidence and is TM-polarized. Parameters of the MPC correspond to the experimentally studied structure. Full magnetization saturation in the external magnetic field is assumed. E y and E || are shown at times when their respective values are maximum. Full size image At normal incidence, only the intensity of the transmitted light is sensitive to the MPC magnetization and there is no Faraday effect, that is, the polarization state of the transmitted light is unaltered. For moderate oblique incidence, the LMPIE remains present and the Faraday effect appears; however, the polarization rotation does not exceed 10 −2 degree. The LMPIE takes largest values at the degenerate resonances of the quasi-TE and quasi-TM modes taking place at the angle of incidence θ =0°, λ =840 nm and θ =±2°, λ=830 nm ( Fig. 4a ). 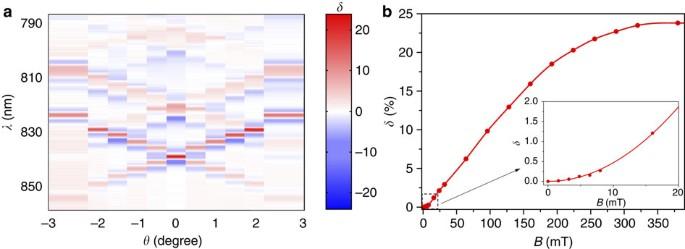Figure 4: Incidence angle and magnetic field dependences of the LMPIE. (a) Contour plot of the incidence angle dependence was measured for TM-polarized illumination andB=320 mT. The LMPIE is largest at the degenerate resonances of the quasi-TE and quasi-TM modes (atθ=0°,λ=840 nm andθ=±2°,λ=830 nm). (b) Magnetic field dependence measured at the highest resonant maximum ofδatλ=840 nm and for TM-polarized illumination hitting the sample normally. The inset shows a close-up of the low magnetic field region demonstrating a quadraticB-field dependence. Figure 4: Incidence angle and magnetic field dependences of the LMPIE. ( a ) Contour plot of the incidence angle dependence was measured for TM-polarized illumination and B =320 mT. The LMPIE is largest at the degenerate resonances of the quasi-TE and quasi-TM modes (at θ =0°, λ =840 nm and θ =±2°, λ =830 nm). ( b ) Magnetic field dependence measured at the highest resonant maximum of δ at λ =840 nm and for TM-polarized illumination hitting the sample normally. The inset shows a close-up of the low magnetic field region demonstrating a quadratic B -field dependence. Full size image The LMPIE is quadratic in the longitudinal magnetization of the MPC, which is supported by a parabolic dependence of the effect on the external magnetic field B for B <30 mT ( Fig. 4b ). Though the saturation occurs for B =360 mT, the LMPIE is quite large even for much smaller magnetic fields. The saturation magnetic field could be diminished down to 10 mT if a magnetic film possessing easy in-plane magnetic anisotropy is used instead. The measured magneto-photonic intensity effect with 24% modulation can be considered giant because its origin is second-order in g . This becomes even more evident if compared with the orientational effect, which is also quadratic in g . For the same bare magnetic film, the orientational effect is negligible: δ ~10 −5 (as calculated for normal incidence and illumination polarized perpendicularly to M ). For metallic ferromagnetics, it reaches maximum values of δ ~10 −3 (Krinchik and Gushchin [33] ). The other MPC sample was based on Bi 2 Dy 1 Fe 4 Ga 1 O 12 magnetic film of thickness h m =873 nm. It has reduced magneto-optical quality (near the quasi-TE-mode resonance at λ =703 nm, g =0.0023 and α =820 cm −1 ) (ref. 35 ). As a result, we measured peak value of δ as 0.85% only. It proves that the LMPIE is crucially dependent on the magneto-optical quality of the magnetic film. Thus, assuming an MPC with a magnetic layer of Bi 3 Fe 5 O 12 having g =0.049 and α =580 cm −1 at 805 nm (ref. 36 ), our calculations demonstrate that the LMPIE can be optimized potentially, leading to δ exceeding 100%. In summary, we demonstrated a new magneto-photonic effect in the longitudinal magnetization configuration for modulating the transparency of the nanostructured sample. Its experimentally observed value δ reaches 24%, which can be considered as a giant value. The modulation level can be increased even further by using materials with better magneto-optical quality, manifesting the relevance of the LMPIE for applications in modern telecommunication devices. Moreover, recent results on the inverse Faraday effect [37] suggest that the LMPIE might be used for all-optical light modulation on sub-nanosecond timescales. On the other hand, the effect of mode switching is of great perspective for active plasmonics and metamaterials [38] , [39] . For example, it might be used in optical transistors to allow efficient control of light propagation in magnetic waveguides through nonlinear interaction [40] with the excited modes of the MPC. Field and dispersion of the electromagnetic modes of the MPC Optical properties of a medium magnetized along the x- axis are characterized by the permittivity tensor : For magnetic dielectrics at optical frequencies, the following inequalities are fulfilled: b<<g<<ɛ 2 , and the permeability μ is close to 1. The constants g and b are linear and quadratic in magnetization, respectively, which can be written in the form b = ag 2 , where a is a magnetization-independent coefficient. Consequently, the contribution of b causes only renormalization of the coefficients in the expressions describing the magneto-optical effect as compared with the case of b =0. Moreover, numerical modelling shows that the contribution of b to the effect is much smaller than the contribution by the g 2 term. That is why in the following analysis we argue in terms of g , assuming that the contribution of b is implicitly taken into account in the corresponding coefficients. Let us first consider the MPC structure in which the metal grating is substituted with a smooth metal. The solutions of the Maxwell’s equations corresponding to waveguide modes are found in the following form (the coordinate axes are shown in Fig. 1 ): in the metal: in the magnetic layer: and in the substrate: where , κ is the mode wavenumber, ɛ 1 and ɛ 3 are dielectric constants of the metal and substrate, respectively, ω is the frequency, c is the speed of light in vacuum, is the unit electric field vector corresponding to polarization denoted by ( j ), and coefficients A i , B i and K i are to be found (see below). Note that the electromagnetic field in the magnetic layer consists of four plane waves with different polarization states, whereas in surrounding media, it contains both TE and TM components. For magnetic media γ and are found from the Fresnel equation: where n denotes the refraction vector n ={ κ ; 0; ± γ ± }. γ ± can be represented as γ ± = γ 2 ±Δ γ ± ( g ), where and Δγ ± is a magneto-optical contribution. Taking into account the boundary conditions for E and H vectors at the metal/magnetic dielectric and magnetic dielectric/substrate interfaces, the following dispersion equation is obtained: where , for the ‘quasi-TM’ modes and η i = γ i for the ‘quasi-TE’ modes, h m is the magnetic layer thickness and Ψ( κ , ω ) is determined by the optical and geometrical parameters of the structure (the expression for Ψ( κ , ω ) is not presented because of its complexity). Excluding some specific cases when , where κ 0 is the mode wavenumber for the demagnetized system (Φ( κ 0 , ω )=0), and taking into account the smallness of g , it follows from equation 8 that the magnetic contribution to κ is quadratic in g : which leads to equation 2: κ = κ 0 (1+ g 2 ), where . The coefficients A i , B i and K i in equation 4 are found by applying boundary conditions for E and H vectors at the two interfaces. Substituting those coefficients in equation 4 reveals that all six components of the electromagnetic field are non-zero, but the admixed components for either of the two modes vanish for g =0. In the linear in g approximation, one can find that the admixed components are proportional to g , whereas the principal components are magnetization independent: for the ‘quasi-TM’ modes: for the ‘quasi-TE’ modes: For given magnetization direction, the functions ( κ , z ) and ( κ , z ) are odd in κ . The explicit formulas for ( κ , z ) and ( κ , z ) have rather complicated form and are not presented here. The presence of the periodic array of slits in the metal layer makes the modes Bloch waves: where U ( x , z ) is a periodic function of x and thus can be expanded in a Fourier series, so that: where m is an integer and d is the grating period. If the slit width is rather small in comparison with the period, then the electromagnetic field distribution for each of the terms in equation 13 is not greatly affected by the slits, as the field is concentrated mostly inside the magnetic layer. It implies that their wavenumbers and therefore the Bloch wavenumber κ can be estimated by equation 2, and equations 10 and 11 also conserve their form for each term in equation 13 in the presence of the slits. At κ =0, equation 13 for the principal components of the quasi-TE and quasi-TM modes takes the form: Applying equations 10 and 11 for each term in equation 14, we derive the expressions for the admixed components: Taking into account that (κ, z ) and (κ, z ) are odd in κ , we come to equation 1. Fabrication The MPC structure was fabricated by the following procedure. The magnetic layer of bismuth-substituted rare-earth iron garnet with composition Bi 2.97 Er 0.03 Fe 4 Al 0.5 Ga 0.5 O 12 was deposited on the gadolinium gallium garnet substrate by rf-magnetron sputtering of the composite 3.2Bi 2 O 3 +4Fe 2 O 3 +0.5Al 2 O 3 +0.5Ga 2 O 3 +0.03Er 2 O 3 oxide target in a 25-mTorr Ar–O2 (4:1) gas mixture at a substrate temperature of 580 °C and rf-power density of 10 W cm −2 . The film synthesis was finalized with in situ postannealing at 550 °C for 10 min at 500 Torr of oxygen pressure [34] . The epitaxial quality of the magnetic film was confirmed by X-ray diffraction patterns. The film shows a uniaxial magnetic anisotropy and a maze-like domain structure of 1 μm typical domain width. The gold grating was fabricated by thermal deposition of a gold layer onto the iron garnet film and subsequent electron beam lithography combined with reactive ion etching by an Ar-ion plasma. Grating period and slit width were determined from atomic force microscopy. All magneto-optical measurements were performed at room temperature. A halogen lamp was used as a white light source. The collimated light was focused on the sample with an achromatic doublet in conjunction with an adjustable iris to reduce the angle of the incoming light cone to <1°. The focused light spot on the sample was about 200 μm in diameter. The polarization of light with respect to the slits was adjusted with a Glan–Thomson prism. Magnetic fields up to 360 mT were applied in the MPC film plane and perpendicularly to the grating slits. The zero-diffraction order-transmitted light was collimated by an achromatic lens and focused on the entrance slit of a spectrograph. The later has linear dispersion of 6.4 nm/mm and is equipped by a charge-coupled device camera, which provides an overall spectral resolution of 0.3 nm. Numerical simulation The electromagnetic modelling was performed using the Rigorous Coupled-Wave Analysis technique extended to the case of gyrotropic materials [41] . The eigenfrequencies of the guided modes of the structure were determined by the scattering-matrix method [42] . For the modelling of the experimentally studied MPC with the Bi 2.97 Er 0.03 Fe 4 Al 0.5 Ga 0.5 O 12 ferromagnetic film, the permittivity ɛ and the gyration g were taken from experiment and from Dzibrou and Grishin [36] (for example, at 840 nm, ɛ =6.440+0.012 i , g =0.015−0.001 i and b =4 × 10 −5 ). Dispersion of both quantities was taken into account. For the permittivity of gold, we used the experimental data from Johnson and Christy [43] . To get optimal correspondence with the experimental data, the gold grating height h gr and slit width r were varied during the electromagnetic modelling within their measurement errors. Best matching was found for h gr =67 nm (experimentally found value of h gr was 65 nm) and r =145 nm (experimentally found value of r was 149 nm). How to cite this article: Belotelov, V. I. et al. Plasmon-mediated magneto-optical transparency. Nat. Commun. 4:2128 doi: 10.1038/ncomms3128 (2013).